Assembly and control of 3D nematic dipolar colloidal crystals Topology has long been considered as an abstract mathematical discipline with little connection to material science. Here we demonstrate that control over spatial and temporal positioning of topological defects allows for the design and assembly of three-dimensional nematic colloidal crystals, giving some unexpected material properties, such as giant electrostriction and collective electro-rotation. Using laser tweezers, we have assembled three-dimensional colloidal crystals made up of 4 μm microspheres in a bulk nematic liquid crystal, implementing a step-by-step protocol, dictated by the orientation of point defects. The three-dimensional colloidal crystals have tetragonal symmetry with antiparallel topological dipoles and exhibit giant electrostriction, shrinking by 25–30% at 0.37 V μm −1 . An external electric field induces a reversible and controllable electro-rotation of the crystal as a whole, with the angle of rotation being ~30° at 0.14 V μm −1 , when using liquid crystal with negative dielectric anisotropy. This demonstrates a new class of electrically highly responsive soft materials. The self- and directed-assembly of micro- or nano-scale objects into robust three-dimensional (3D) structures with predetermined architecture and functionality is one of the major goals of material science. Geometrically regular 3D micro-structures from dielectric objects are called photonic crystals [1] and have attracted immense interest because of their ability to guide and control light at a microscale. Fabrication of photonic crystals has been approached using a variety of techniques, such as directed colloidal crystallization on patterned surfaces [2] , micromanipulation using micro-mechanical [3] , laser or optoelectronic tweezers [4] , colloidal self-assembly via DNA hybridization [5] and so on. The aim is to control the pair-interaction forces between the particles to such a degree that thermally stable 3D micro- and nanostructures with predetermined architectures can be assembled. Nematic liquid crystals (LCs) mediate anisotropic forces between the colloidal particles that could potentially be used for colloidal 3D self-assembly and have therefore attracted significant interest from both theoretical and experimental aspects [6] , [7] , [8] , [9] , [10] . These effective forces are caused by the elastic deformation of the nematic LC, and can be much more complex than the forces between electric charges, mediated by an electromagnetic field. At the heart of colloidal interactions in LCs is the tensorial nature of the ordering field in LCs, which is ultimately mediating the colloidal interactions. Because of the inherent complexity of this interacting field, the topology of the field becomes important for colloidal interactions. It is responsible for the striking emergence of topological-defect-mediated interactions in two-dimensional (2D) colloids, such as the assembly of 2D nematic colloidal crystals by singular topological point defects [11] , colloidal interactions mediated by colloidal entanglement [12] , [13] , where knotted and linked topological defect loops could form colloidal knots and links of arbitrary complexity [14] . Till now and in most cases, nematic colloidal interactions have been experimentally studied, controlled and exploited in two dimensions, although in some cases the thickness of the nematic layer was much larger compared with the particle size [15] , [16] , including the study of confinement effects on pair interaction [17] . The main reason is that optical microscopy used in colloidal studies provides an effective 2D information about the system at a given moment of time so a single microscopic photograph contains information that is integrated along the light path. The optical microscopy observations therefore reveal just a particular projection of the full 3D interaction map between the colloidal particles. The confocal microscopy (including fluorescent confocal polarizing microscopy, FCPM [18] ) provides truly 3D information about the investigated system and has been used successfully for fast imaging in water-based colloids [19] . However, this method is too slow for real-time 3D imaging and recovery of colloidal pair interactions in LCs because of the small amount of added fluorescent dye and low level of fluorescent light emission. At the same time it was generally understood from the basic symmetry considerations that the elastic interaction between colloidal particles is not limited to two dimensions. There were predictions [20] as well as experimental studies reporting the formation of irregular 3D colloidal clusters in nematic LCs [21] , [22] . Recently, computer simulations were used to study colloidal interactions and regular clusters in LCs in full three dimensions [23] . Here we explore the nematic colloidal interactions in 3D by studying and controlling the forces between colloidal particles with normal surface anchoring in bulk nematic LCs using the laser tweezers. The conservation of the topological charge ensures that each colloidal particle in the bulk nematic LC is accompanied by a topological point defect, thus forming a topological dipole with a dipolar symmetry of the elastically deformed nematic LC. We observe that like with electric dipoles, the topological dipoles in 3D interact via the long-range elastic deformation of the director field, resulting in several thousands of k B T interaction energy per micrometer-sized particle. Laser tweezers are used to manipulate and control the single colloids as well as their chains and small 3D crystals and finally direct the colloidal assembly into well-ordered 3D colloidal crystals of elastic dipoles. Visualization of the assembling is provided with a series of microscopy movies of the assembly process (see Supplementary Information and Supplementary Videos ). By using FCPM we observe that the symmetry of the assembled 3D dipolar colloidal crystal unit cell is tetragonal and is in good agreement with Landau-de Gennes theory. We demonstrate that the application of an external electric field along the dipoles induces a significant and controllable shrinkage of the 3D dipolar colloidal crystal when dielectric anisotropy of the host LC material is positive. When we use a LC with negative dielectric anisotropy, we observe spatial rotation of the 3D colloidal crystal as a whole, which is directly and reversibly controlled by the strength of the electric field. Quasi-2D checkerboard dipolar colloidal structure Optical microscope images of individual 2.32 μm silica microspheres in ~10 μm-thick homeotropic layer of 5CB nematic LC are shown in ( Fig. 1a ). The microspheres clearly appear in two different forms, which correspond to either an up or down orientation of their topological dipoles, as explained in Supplementary Fig. S1 and Supplementary Note 1 . Besides individual and isolated colloidal particles, we also observe spontaneously formed colloidal clusters with a quasi-2D square lattice, with particles shifted up or down in rectangular sub-lattices, as shown in ( Fig. 1c ). The particles in the quasi-2D square lattice are arranged in a ‘checkerboard-like’ manner: each brighter particle has four darker particles as direct neighbours and vice versa. Such an arrangement clearly suggests that brighter and darker particles have opposite directions of their topological dipoles. This arrangement of the dipoles minimizes the free energy of the colloidal lattice and is similar to the antiferromagnetic interaction of magnetic dipoles [24] . The confocal cross-section image of the checkerboard colloidal structure is shown in ( Fig. 1d ) and confirms the alternating orientation of the topological dipoles. Moreover, the vertical positions of the centres of mass of the colloidal particles also alternate between neighbouring particles: lower particles have defects above and upper particles have defects below (see the analysis in Supplementary Note 1 , illustrated with Supplementary Figs S2, S3 and S4 ). 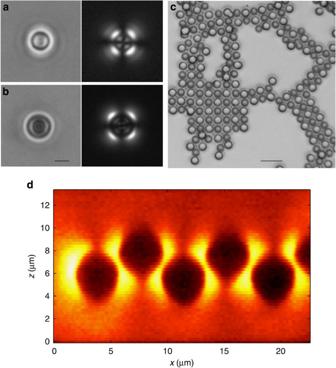Figure 1: Colloidal particles with dipolar symmetry in a thin layer of a nematic liquid crystal. (a,b) Microscopic images of 2.32 μm dipolar silica microspheres in the homeotropic cell filled with 5CB nematic liquid crystal. In (a), the topological point defect is above the microsphere, in (b), the defect is below it. Left panels are taken without polarizers, right panels are taken between crossed polarizers. Scale bar, 2 μm. (c) Quasi-2D checkerboard structure formed by 4.32 μm silica particles in ~10 μm-thick homeotropic cell filled with ZLI-2806. The lattice was observed with completely open condenser aperture diaphragm enhancing the ‘checkerboard’-like look of the crystal. No polarizers were used. Scale bar, 10 μm. (d) A vertical cross-section of a quasi-2D checkerboard colloidal crystal of 4 μm colloidal particles, obtained from confocal microscope imaging of a structure like in (c). The alternating arrangement of the microspheres with topological defects above and below them is clearly seen. The defects are not resolved in this image, they are located in the points where the two bright lobes that encircle each particle come together. More details are in Supplementary Note 1. Figure 1: Colloidal particles with dipolar symmetry in a thin layer of a nematic liquid crystal. ( a , b ) Microscopic images of 2.32 μm dipolar silica microspheres in the homeotropic cell filled with 5CB nematic liquid crystal. In ( a ), the topological point defect is above the microsphere, in ( b ), the defect is below it. Left panels are taken without polarizers, right panels are taken between crossed polarizers. Scale bar, 2 μm. ( c ) Quasi-2D checkerboard structure formed by 4.32 μm silica particles in ~10 μm-thick homeotropic cell filled with ZLI-2806. The lattice was observed with completely open condenser aperture diaphragm enhancing the ‘checkerboard’-like look of the crystal. No polarizers were used. Scale bar, 10 μm. ( d ) A vertical cross-section of a quasi-2D checkerboard colloidal crystal of 4 μm colloidal particles, obtained from confocal microscope imaging of a structure like in ( c ). The alternating arrangement of the microspheres with topological defects above and below them is clearly seen. The defects are not resolved in this image, they are located in the points where the two bright lobes that encircle each particle come together. More details are in Supplementary Note 1. Full size image Laser-tweezers assembly of a 3D dipolar colloidal crystal We now use the up/down orientation of the isolated topological dipoles in homeotropic LC cells to assemble up/down oriented dipolar colloidal chains of microspheres in a bulk LC (see Supplementary Movie S1 ). It is known [7] that like with electric dipoles, dipolar nematic colloids readily form colloidal chains along the LC director in planar cells and they also do so in homeotropic cells. In this case, the chains are observed along their direction and we can distinguish the number of particles in the chain, because more particles create an effectively thicker, distorted, birefringent volume of LC. Longer chains therefore appear brighter and larger compared with single particles, as illustrated in ( Fig. 2a ). 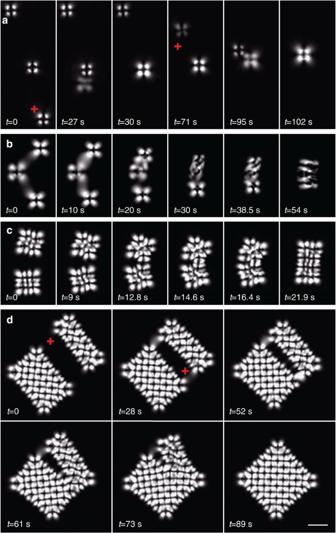Figure 2: Laser-tweezers assembly of a 3D dipolar colloidal crystal observed under crossed polarizers. (a) Three isolated colloidal particles of 4 μm diameter in the ZLI-2806-filled homeotropic cell of ~25 μm thickness appear as bright objects with a dark cross in the centre. Using laser tweezers, one particle is brought close to the other and they spontaneously form a chain of two particles in a direction perpendicular to the plane of the image. The pair appears like a single but larger and brighter particle (3rd image from the left). The third particle is brought to the couple and it spontaneously forms a dipolar colloidal chain of three particles on top of each other. (b) Three chains, each made of three dipolar particles, are brought close to each other and they start to assemble into a frustrated colloidal trio. Note the tilting of the chains. (c) Two colloidal blocks of 2 × 2 × 3 particles self-assemble into 2 × 4 × 3 blocks. (d) Colloidal blocks of 2 × 6 × 3 and 4 × 6 × 3 particles assemble into the final 6 × 6 × 3 dipolar colloidal crystal. The assembly at the initial stage was guided by the laser tweezers until blocks started to attract themselves. Scale bar, 10 μm. In all images, the small red cross is the optical trap, used to direct the colloidal assembly. Figure 2: Laser-tweezers assembly of a 3D dipolar colloidal crystal observed under crossed polarizers. ( a ) Three isolated colloidal particles of 4 μm diameter in the ZLI-2806-filled homeotropic cell of ~25 μm thickness appear as bright objects with a dark cross in the centre. Using laser tweezers, one particle is brought close to the other and they spontaneously form a chain of two particles in a direction perpendicular to the plane of the image. The pair appears like a single but larger and brighter particle (3rd image from the left). The third particle is brought to the couple and it spontaneously forms a dipolar colloidal chain of three particles on top of each other. ( b ) Three chains, each made of three dipolar particles, are brought close to each other and they start to assemble into a frustrated colloidal trio. Note the tilting of the chains. ( c ) Two colloidal blocks of 2 × 2 × 3 particles self-assemble into 2 × 4 × 3 blocks. ( d ) Colloidal blocks of 2 × 6 × 3 and 4 × 6 × 3 particles assemble into the final 6 × 6 × 3 dipolar colloidal crystal. The assembly at the initial stage was guided by the laser tweezers until blocks started to attract themselves. Scale bar, 10 μm. In all images, the small red cross is the optical trap, used to direct the colloidal assembly. Full size image We use cells of such thickness (usually around ≈25 μm) that three 4 μm colloidal-microsphere chains with one of the two directions of their topological dipoles can easily be floating in a LC without touching the cell’s surfaces, which mimics bulk 3D colloidal assembly. Bigger colloidal clusters are assembled from individual three-particles-long colloidal chains using the laser tweezers. When the three chains of three particles are brought together close enough for them to strongly attract to each other, laser tweezers are switched off and the particles form a frustrated, V-shaped colloidal trio, as shown in ( Fig. 2b ) and Supplementary movie S2 . This is actually the most difficult step in the assembly of 3D nematic colloidal crystals, as a trio of colloidal chains seems to prefer a non-planar tilted configuration, which is obviously a result of the topological frustration. This three-body topological frustration is also observed in the experiments with planar nematic cells (see Supplementary Figs S5, S6, S7 and Supplementary Note 2 ) and is analogous to the orientational frustration in spin systems, such as the Kagome lattice [24] , where a pair of spins has the lowest energy in the antiparallel orientation, but the third spin on the lattice is frustrated in its orientation as it cannot simultaneously be up and down. However, this frustration is released when a properly oriented fourth colloidal chain is brought closer with the laser tweezers, and a final colloidal block of four chains of microspheres is formed, as shown in the first panel of ( Fig. 2c ). After building several isolated and well-ordered blocks of 2 × 2 × 3 colloidal particles, a bigger, 3D, dipolar, colloidal crystal can be easily assembled by guiding and directing the self-assembly of the colloidal blocks into the minimum-energy positions (see Supplementary Movies S3, S4 and S5 ). Figure 2c shows an example of the self-assembly of two colloidal blocks of 2 × 2 × 3 particles into a larger block of 2 × 4 × 3 particles. The two blocks are positioned with the laser tweezers in a proper orientation and then released. They are spontaneously attracted to each other by elastic forces over a separation of more than 10 μm. These blocks are then brought together with laser tweezers, and self-assemble into even larger 3D colloidal blocks. Figure 2d shows video snapshots of the assembly of the biggest 3D colloidal crystal of 6 × 6 × 3 particles that was produced by merging a 2 × 6 × 3 colloidal block and a 4 × 6 × 3 colloidal block. The colloidal crystals are very robust and can be dragged with the laser tweezers without causing any permanent damage, as illustrated in Supplementary movie S7 . The arrangement of the colloidal particles in the 3D dipolar colloidal crystal of 6 × 6 × 3 particles is determined by FCPM [18] and is shown in Fig. 3 . It is clear from the subsequent FCPM cross-sections, focusing on subsequent crystal layers ( Fig. 3a ) that the colloidal particles are arranged in a regular tetragonal Bravais lattice with basis, with lattice constants A =(6.4±0.2)μm, B =(4.6±0.4)μm, or in units of particle radius A =(3.2±0.1) R , B =(2.3±0.2) R , and were determined directly from the recorded FCPM images. The 3D representation of the colloidal crystal, as reconstructed from the FCPM images is shown in Fig. 3b (see also Supplementary movie S6 ) and clearly presents the 3D tetragonal symmetry of the nematic colloidal crystal. The central colloidal particle is positioned at the basis vector corresponding to Ψ=(1.3±0.1) R (see Fig. 3e ), which indicates the elevation of the particle in the elementary cell. 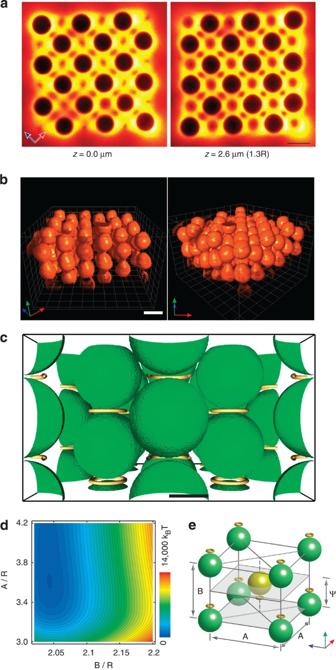Figure 3: Structure of a 3D dipolar nematic colloidal crystal. (a) Fluorescent confocal polarizing microscopy images of two horizontal cross-sections of a 3D, 6 × 6 × 3 dipolar colloidal crystal, assembled from 4 μm diameter colloidal particles in the homeotropic aligned nematic liquid crystal ZLI-2806. The images were acquired by refocusing along thez-axis direction by 2.6 μm . Scale bar, 5 μm. (b) The 3D representation of the fluorescent confocal polarizing microscopy image of a 6 × 6 × 3 3D dipolar colloidal crystal. Here, the fluorescence intensity was inverted to show the in-plane arrangement of the particles in the XY, YZ and XZ planes. Scale bar, 5 μm. (c) Numerical simulation of a 3D dipolar nematic colloidal crystal. Point topological defect opened into small loops, somewhat larger as observed in experiments, and are visualized as iso-surfaces of fixed nematic degree of orderS. Scale bar, 1 μm. (d) Free energy of one colloidal crystal unit cell as a function of the lattice constants A and B in units of particle radiusR. (e) Schematic drawing of the crystal structure showing the tetragonal Bravais lattice with basis. Figure 3: Structure of a 3D dipolar nematic colloidal crystal. ( a ) Fluorescent confocal polarizing microscopy images of two horizontal cross-sections of a 3D, 6 × 6 × 3 dipolar colloidal crystal, assembled from 4 μm diameter colloidal particles in the homeotropic aligned nematic liquid crystal ZLI-2806. The images were acquired by refocusing along the z -axis direction by 2.6 μm . Scale bar, 5 μm. ( b ) The 3D representation of the fluorescent confocal polarizing microscopy image of a 6 × 6 × 3 3D dipolar colloidal crystal. Here, the fluorescence intensity was inverted to show the in-plane arrangement of the particles in the XY, YZ and XZ planes. Scale bar, 5 μm. ( c ) Numerical simulation of a 3D dipolar nematic colloidal crystal. Point topological defect opened into small loops, somewhat larger as observed in experiments, and are visualized as iso-surfaces of fixed nematic degree of order S . Scale bar, 1 μm. ( d ) Free energy of one colloidal crystal unit cell as a function of the lattice constants A and B in units of particle radius R . ( e ) Schematic drawing of the crystal structure showing the tetragonal Bravais lattice with basis. Full size image The stability and structure of the 3D dipolar nematic colloidal crystals were analysed within the Landau-de Gennes theory, studying both the structure of the colloidal lattice formed by the microspheres and the ordering of the underlying nematic fluid. The total free energy was minimized numerically in a unit cell of variable size and with variable positions of the (two) colloidal particles, based on the order-parameter tensor Q ij and constructed from the elasticity, the variation of the order, and the surface anchoring [25] , [26] . The topology of the field was imprinted into the colloidal structure via the initial conditions of Q ij , using the superposition of the dipolar Ansätze, locally, around each individual particle. The results are shown in Fig. 3c . Theory predicts that the stable colloidal crystalline structure consists of antiparallel dipolar chains that constitute a tetragonal, colloidal crystal with a basis (see the sketch in Fig. 3e )—as was indeed observed in the experiments. In the calculations, the topological −1 hyperbolic hedgehog defects opened into small rings, more so than in the experiments, yet they retained the dipolar symmetry of the director field around the individual particles. Calculating the total free energy of the colloidal crystalline unit cell as a function of the lattice constants A and B shows that the colloidal crystal is strongly bound along the direction of the dipolar chains, but it is weaker in the direction perpendicular to the chains ( Fig. 3d ). Interestingly, upon expanding or shrinking the unit cell of the colloidal crystal, we find the variation in the elevation Ψ of the middle particle in the elementary cell of the colloidal crystal is as strong as ~10%, indicating a large susceptibility to manipulation with electrostriction. The assembly of 3D colloidal crystals reveals the important role of finite size. The director field of the individual dipolar chains, as the elementary building block of the crystal, is asymmetric—one end of the chain ends with the hyperbolic point defects, whereas the other ends with a particle. And when assembling multiple dipolar chains into the crystal these ends of the chains create locally net elastic torques [27] that cause tilting of the crystal as a whole, as observed in both the experiments (see Fig. 2b ) and in the numerical modelling. Depending on the specific, finite size of the crystal, that is, the number of x × y chains, the chains of the crystal are oriented along the direction of the undistorted director (along z ) or they are tilted. This orientational symmetry/asymmetry is clearly seen in the 2 × 2-chains colloidal block, where it can be characterized by two mutually perpendicular symmetry planes of the nematic profile. The symmetry planes correspond to no-net-torque conditions in two perpendicular directions and the 2 × 2 block remains untilted. In contrast, for example, in a 2 × 3 or 3 × 2-chains block, one symmetry plane is lost and the whole-colloidal structure tilts. Besides tilting, another relevant finite-size effect is the confinement of the nematic profile by the cell in which the assembly is performed. Effectively, the confinement affects the interparticle potentials between the chains, and this can cause weak bending of the chains close to the confining surfaces, that is, locally shorter lattice constants. It is known that nematic LCs are very sensitive to external electric fields because LC molecules with a positive dielectric anisotropy (Δ ε >0) tend to align collectively in the direction of the external field, while in the case of a negative dielectric anisotropy (Δ ε <0) they tend to align perpendicular to the field [25] . When the electric field is applied to a LC with colloidal particles the equilibrium molecular orientation configuration around a single particle is no longer determined just by the particle itself. The stronger the applied field is, the stronger the effect it has on the surrounding LC molecules and the effect of the particle decreases. This field-induced reorientation of the LC molecules around the colloidal particles changes the elastic forces between the particles, resulting in the field dependence of the lattice constant of the colloidal crystal. It was shown that the lattice constants of a 2D-dipolar crystal in a planar nematic LC cell change anisotropically under the action of an electric field that is applied perpendicular to the crystal [28] . We have measured the electric-field response of the 3D dipolar nematic colloidal crystal for two different nematic LCs with a positive and negative dielectric anisotropy. In both cases the electric field was applied through transparent ITO electrodes in a direction perpendicular to the glass surfaces of the measuring cell. When an electric field is applied to the 3D dipolar colloidal crystal assembled in an E7 LC material with Δ ε >0, the crystal shrinks dramatically along all the basis directions, as demonstrated in Fig. 4a . This shrinkage is controllable and fully reversible and the lattice constant changes by ~25−30% at 0.37 V μm −1 , see Fig. 4b , in several hundreds of milliseconds. It is also clear from Fig. 4a that the region of the deformed LC director field around each chain shrinks with the increasing electric field. Far away from the particles the orientation of the LC molecules does not change because they are already oriented along the direction of the applied field. The applied field therefore only acts on those LC molecules that were rotated away from the global homeotropic sample orientation by the particles, thus shortening the effective interaction range of the neighbouring chains and decreasing its absolute magnitude. By considering the interaction of five chains that belong to the single elementary cell presented in Fig. 3e one can see that the peripheral chains repel each other because they have the same dipole orientation. Only their attraction to the central chain with an opposite dipole direction stabilizes the elementary cell. These two interactions change under an electric field and become more localized because of the electric-field-induced alignment of the LC molecules, so the repulsive components in the single elementary cell can now be balanced by weaker attraction components at smaller distances, which leads to shrinking of the elementary cell. 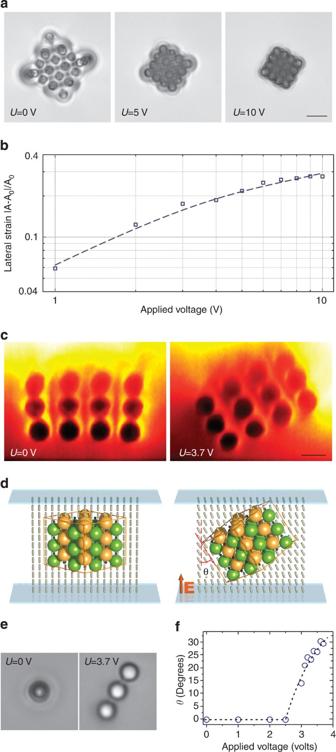Figure 4: Electric-field-induced shrinkage and rotation of a 3D dipolar nematic colloidal crystal. (a) 4 × 4 × 3 dipolar nematic colloidal crystal made of 4.32 μm colloids in E7 shrinks under an applied electric field. The dielectric anisotropy of the host LC is positive, Δε>0. Scale bar, 10 μm. (b) Relative lateral shrinkage, seeFig. 3e) as a function of applied voltage for 3D crystal in E7 (Δε>0) nematic liquid crystal mixture. The electric field (f=1 kHz) is applied along theBaxis of the elementary cell. Dashed line is guide to the eyes. (c) Fluorescent confocal polarizing microscopy images of electric-field-induced rotation of a 3D, 4 × 4 × 3 dipolar nematic colloidal crystal in a ZLI-2806 liquid crystal with negative dielectric anisotropy, Δε<0. Scale bar, 5 μm. (d) Schematic views of 3D dipolar crystal and liquid crystal configuration without field (left) and after electric field is applied, inducing rotation of 3D nematic colloidal crystal as a whole (right). The crystal follows the liquid crystal molecules, which tend to align perpendicular to the field because of their negative dielectric anisotropy. (e) Microscope images of electric-field-induced rotation of a single colloidal chain in ZLI-2806 liquid crystal. The chain in the left panel points into the panel and is rotated from this direction by the field. (f) Angle of rotation of a colloidal crystal as a function of applied electric field. Figure 4: Electric-field-induced shrinkage and rotation of a 3D dipolar nematic colloidal crystal. ( a ) 4 × 4 × 3 dipolar nematic colloidal crystal made of 4.32 μm colloids in E7 shrinks under an applied electric field. The dielectric anisotropy of the host LC is positive, Δ ε >0. Scale bar, 10 μm. ( b ) Relative lateral shrinkage , see Fig. 3e ) as a function of applied voltage for 3D crystal in E7 (Δ ε >0) nematic liquid crystal mixture. The electric field ( f =1 kHz) is applied along the B axis of the elementary cell. Dashed line is guide to the eyes. ( c ) Fluorescent confocal polarizing microscopy images of electric-field-induced rotation of a 3D, 4 × 4 × 3 dipolar nematic colloidal crystal in a ZLI-2806 liquid crystal with negative dielectric anisotropy, Δ ε <0. Scale bar, 5 μm. ( d ) Schematic views of 3D dipolar crystal and liquid crystal configuration without field (left) and after electric field is applied, inducing rotation of 3D nematic colloidal crystal as a whole (right). The crystal follows the liquid crystal molecules, which tend to align perpendicular to the field because of their negative dielectric anisotropy. ( e ) Microscope images of electric-field-induced rotation of a single colloidal chain in ZLI-2806 liquid crystal. The chain in the left panel points into the panel and is rotated from this direction by the field. ( f ) Angle of rotation of a colloidal crystal as a function of applied electric field. Full size image However, when the 3D dipolar crystal is assembled in a nematic LC with Δ ε <0 (ZLI-2806), the response to the electric field is strikingly different. Instead of the electric-field-induced shrinkage observed for the positive dielectric anisotropy, the 3D colloidal crystal rotates as a whole by a distinct angle θ , preserving its shape, as illustrated by the FCPM images in Fig. 4c and Supplementary Movie S8 . The rotation is due to the different response of the negative dielectric anisotropy nematic LC to the applied field. In the material with Δ ε <0, the initial global orientation in the sample is also homeotropic and hence along the applied electric field direction. When the applied field reaches the threshold magnitude for the Freedericksz transition [25] , the LC molecules start to rotate away from the field direction, tending to align perpendicular to it, as illustrated in Fig. 4d . Such a global reorientation of the LC molecules is a collective effect and occurs throughout the whole cell. The colloidal crystal remains in the initial orientation until the applied field reaches the Fredericksz threshold voltage (~2.5 V, see Fig. 4f ) and rotates as a whole when the field is above the Fredericksz threshold voltage (see Supplementary Fig. S8 and Supplementary Note 3 ). The electric-field-induced rotation is also observable for a chain of three colloidal particles ( Fig. 4e ). The tilting angle depends on the magnitude of the electric field, which is relatively high and the crystal rotates by as much as ~30° in an electric field of only 0.14 V μm −1 . We find that the lattice constant B, determining the positions of colloidal particles along the dipolar chains, is practically independent of the voltage, as shown in Supplementary Fig. S9 . The lateral lattice constant A(U) is practically voltage-independent up to the Fredericksz transition, where the reorientation is accompanied by sudden shrinkage, followed by gradual expansion to the original value. The electrostriction and electro-rotation of the 3D crystal can be combined in a dual-frequency nematic LC that changes the sign of its dielectric anisotropy at a certain frequency. The electric-field-induced rotation of individual solid platelets in the nematic LC was observed by Lapointe et al. [29] Our work on the assembly of 3D colloidal crystals in a nematic LC clearly demonstrates the importance of topological constraints for composite soft-matter materials, such as the spatial and temporal sequential positioning of topological defects. Although in our case the topology of the underlying complex fluid providing the topological defects is rather simple, it is important for tailoring, designing and assembling 3D nematic colloidal crystals. It is also responsible for novel and unexpected material properties that are not realizable in conventional water-based colloids. We have not only shown that 3D nematic colloidal crystals exhibit giant electrostriction, we have also demonstrated a collective electro-rotation of a 3D crystal in an external electric field. We believe that the concept of the defect tailoring of materials could be down-scaled to nano-colloidal dispersions in LCs and other complex soft-matter materials that feature novel material properties. Cells The experiments were performed with nematic colloidal dispersions confined to cells that were assembled from thoroughly cleaned glass slides of 18 × 18 mm 2 size with transparent indium-tin oxide (ITO) electrodes. The ITO was covered with a thin layer of SE-1211 polyimide (Nissan chemicals) or a monolayer of DMOAP (octadecyldimethyl (3-trimethoxysilylpropyl) ammonium chloride, ABCR GmbH) to induce normal (homeotropic) anchoring of the LC molecules at the ITO surface. The thickness of the LC in the gap between the glass plates was controlled by mylar spacers of 10 or 25 μm thickness. Usually cells were made of 1 mm thick glass slides but for confocal experiments we used 170 μm thick ITO covered glass (supplied by SPI) as one of the substrates due to short working distance of the × 100 oil immersion microscope objective. Particles The experiments were performed with silica microspheres of 2.32 and 4.32 μm diameter (Bangs labs), or 4 μm silica-polymer resin composite microspheres (Licristar 40, Merck Inc.). In all cases, the particles were covered with a DMOAP monolayer to induce a perpendicular orientation of the LC molecules on their surfaces. Details of the surface treatment procedure can be found in [30] . The colloidal dispersion was prepared by mixing 1−2 wt% of colloidal particles into the nematic LC and then introduced into the glass cell by capillary forces. LC materials Four different nematic LC materials were used in our experiments, which have different optical and dielectric anisotropies. 5CB (4′-n-pentyl,4-cyanobiphenyl) is a standard single component nematic with high birefringence (Δ n ≈0.2) and positive dielectric anisotropy (Nematel). E7 is a standard, high birefringence nematic LC with Δ n ≈0.2 and positive dielectric anisotropy Δ ε> 0. ZLI-2806 (Merck Inc.) is a low-birefringence nematic LC mixture with n o =1.48, n e =1.52, Δ n ≈0.04. This material also has a negative dielectric anisotropy Δ ε< −4.8. MLC-2048 (Merck Inc.) is a dual-frequency nematic mixture with high birefringence Δ n ≈0.22. The crossover frequency, where the dielectric anisotropy changes sign from to is f cr ≈20 kHz. Laser tweezers Colloidal particles in the nematic LC were manipulated using the laser tweezers setup built around an inverted optical microscope (Nikon TE-2000) with 1064, nm CW laser controlled by a pair of acousto-optic deflectors (AOD, Aresis). Typical laser power was ~50 mW at the focal point and allowed for effective colloidal manipulation. Water immersion × 60 objective with NA=1.0 was used both for trapping and observation of the colloidal particles during the assembly procedure. Fluorescent Confocal Polarizing Microscopy (FCPM) In order to visualize director distribution around colloidal particles in the quasi-3D structure and recover spatial arrangement of the colloids in 3D dipolar crystals we used FCPM [18] setup built around TE-2000 inverted Nikon microscope with CARV-II spinning disc confocal module (BD Biosciences) and × 100 oil-immersion objective (Nikon Plan Apo, NA=1.4, working distance 0.17 mm). To perform fluorescence confocal polarizing microscopy, we have added ~0.01 wt% of ‘Nile Red’ dye (Sigma Aldrich) to the low-birefringence nematic LC mixture ZLI-2806. This dye has anisometric (elongated) molecules so when dissolved in calamitic LC they become aligned by LC due to ‘guest-host’ effect. In this case light-absorption as well as the light emission of the dye depend on the relative orientation of excitation and detection polarization direction and orientation of the dye (and hence LC) molecules [18] . This allows us to correlate the detected polarized fluorescence intensity with the local orientation of the nematic LC and determine locations of the colloidal particles which appear as dark non-emitting areas (holes in LC) on confocal images. In order to achieve good depth resolution and to be able to see beyond the very first layer of colloids in the 3D crystal it is extremely important to have minimal refractive index difference between the LC matrix and colloidal particles. For our confocal experiments we used 4.0 μm particles mentioned above as their refractive index nearly matches that of the ZLI-2806 LC matrix. Along with low birefringence of the matrix itself this allowed us to focus deep into sample and determine orientation of LC around the particles and locations of particles themselves in the 3D crystals we have built. Although the LC matrix has very low birefringence it still causes light de-focusing and confocal image degradation when focused deep into sample. But in our experiments on focus depth up to≈10–12 μm for quasi-3D structures and ≈18–22 μm for 3D dipolar crystals we still were able to obtain good images. Intensity variations on the confocal images recorded with applied electrical field appear because of non-uniform orientation of the LC in the cell. In case of Quasi-3D structure both top and bottom sub-layers are clearly visible and experimental and calculated LC orientation around the particles nicely match each other (See SI, section A). Landau-de Gennes modelling of 3D nematic colloids Mean field Landau-de Gennes approach based upon the tensor order parameter, Q ij is used to model the 3D nematic colloids. This approach constructs the phenomenological free energy F , which naturally accounts for effective elasticity of the LC, variations in the magnitude of the order, and possible biaxiality. We are interested in the assembly of homeotropic few micron-sized spherical particles, within a 3D unit cell. Elastic constants of 5CB nematic LC, used in the experiments, differ for at most of several 10% [31] ; therefore, one elastic constant approximation constant is used. The total free energy F reads: Here, summation over repeated indices is assumed, L is the single elastic constant, A , B and C are nematic material parameters, W is the surface anchoring strength and determines the preferential orientation and order at the colloidal surfaces. First two terms in equation 1 are integrated over LC volume, whereas the last term is integrated over the surfaces of the particles. We find the aimed-at colloidal nematic structure, by minimizing the total free energy. The minimization corresponds to solving a system of coupled partial differential equations with appropriate boundary conditions. Here, we use an explicit Euler finite difference relaxation algorithm on a cubic mesh, applied in a simulation box that is periodic in three spatial dimensions, with total of two particles. To achieve the desired nematic colloidal structure, initial conditions are chosen according to local elastic dipoles [27] . The surface of each particle is defined by the set of mesh points contained within a spherical shell with thickness equal to the mesh resolution. For computational efficiency, the effects of fluid flow are neglected in the relaxational dynamics as these are not expected to effect the equilibrium configurations. Material parameters are chosen to correspond to the experiments with 5CB and are taken to be: L =4.0 × 10 −11 N, a =−0.172 × 10 6 J m −3 , b =−2.12 × 10 6 J m −3 , c =1.73 × 10 6 J m −3 , W =1.0 × 10 −2 J m −2 , and the diameter of the colloidal particles d =2.0 μm. How to cite this article: Nych, A. et al. Assembly and Control of 3D Nematic Dipolar Colloidal Crystals. Nat. Commun. 4:1489 doi: 10.1038/ncomms2486 (2013).